Information processing using a single dynamical node as complex system Novel methods for information processing are highly desired in our information-driven society. Inspired by the brain's ability to process information, the recently introduced paradigm known as 'reservoir computing' shows that complex networks can efficiently perform computation. Here we introduce a novel architecture that reduces the usually required large number of elements to a single nonlinear node with delayed feedback. Through an electronic implementation, we experimentally and numerically demonstrate excellent performance in a speech recognition benchmark. Complementary numerical studies also show excellent performance for a time series prediction benchmark. These results prove that delay-dynamical systems, even in their simplest manifestation, can perform efficient information processing. This finding paves the way to feasible and resource-efficient technological implementations of reservoir computing. Nonlinear systems with delayed feedback and/or delayed coupling, often simply put as 'delay systems', are a class of dynamical systems that have attracted considerable attention, both because of their fundamental interest and because they arise in a variety of real-life systems [1] . It has been shown that delay has an ambivalent impact on the dynamical behaviour of systems, either stabilizing or destabilizing them [2] . Often it is sufficient to tune a single parameter (for example, the feedback strength) to access a variety of behaviours, ranging from stable via periodic and quasi-periodic oscillations to deterministic chaos [3] . From the point of view of applications, the dynamics of delay systems is gaining more and more interest. While initially it was considered more as a nuisance, it is now viewed as a resource that can be beneficially exploited. One of the simplest possible delay systems consists of a single nonlinear node whose dynamics is influenced by its own output a time τ in the past. Such a system is easy to implement, because it comprises only two elements, a nonlinear node and a delay loop. A well-studied example is found in optics: a semiconductor laser whose output light is fed back to the laser by an external mirror at a certain distance [4] . In this article, we demonstrate how the rich dynamical properties of delay systems can be beneficially employed for processing time-dependent signals, by appropriately modifying the concept of reservoir computing. Reservoir computing (RC) [5] , [6] , [7] , [8] , [9] , [10] is a recently introduced, bio-inspired, machine-learning paradigm that exhibits state-of-the-art performance for processing empirical data. Tasks, which are deemed computationally hard, such as chaotic time series prediction [7] , or speech recognition [11] , [12] , amongst others, can be successfully performed. The main inspiration underlying RC is the insight that the brain processes information generating patterns of transient neuronal activity excited by input sensory signals [13] . Therefore, RC is mimicking neuronal networks. 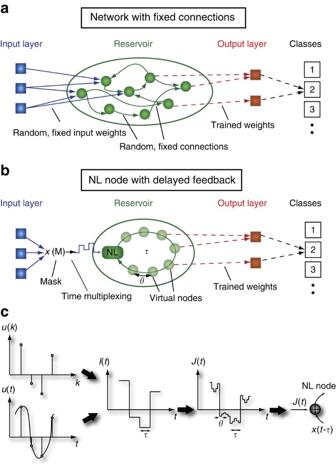Figure 1: Sketch of RC schemes. (a) Classical RC scheme. The input is coupled into the reservoir via a randomly connected input layer to the N nodes in the reservoir. The connections between reservoir nodes are randomly chosen and kept fixed, that is, the reservoir is left untrained. The reservoir's transient dynamical response is read out by an output layer, which are linear weighted sums of the reservoir node statesxi(t). The outputthus has the form. The coefficientswiof the sum are optimized in the training procedure to best project onto the target classes. (b) Scheme of RC utilizing a nonlinear node with delayed feedback. A reservoir is obtained by dividing the delay loop intoNintervals and using time multiplexing. The input states are sampled and held for a durationτ, whereτis the delay in the feedback loop. For any timet0, the input state is multiplied with a mask, resulting in a temporal input streamJ(t) that is added to the delayed state of the reservoirx(t−τ) and then fed into the nonlinear node. The output nodes are linear weighted sums of the tapped states in the delay line given by. (c) Scheme of the input data preparation and masking procedure. A time-continuous input streamu(t) or time-discrete inputu(k) undergoes a sample and hold operation, resulting in a streamI(t) that is constant during one delay intervalτbefore it is updated. The random matrixMdefines the coupling weights from the input layer to the virtual nodes. The temporal input sequence, feeding the input stream to the virtual nodes, is then given byJ(t)=M×I(t). Traditional RC implementations are generally composed of three distinct parts: an input layer, the reservoir and an output layer, as illustrated in Figure 1a . The input layer feeds the input signals to the reservoir via fixed random weight connections. The reservoir usually consists of a large number of randomly interconnected nonlinear nodes, constituting a recurrent network, that is, a network that has internal feedback loops. Under the influence of input signals, the network exhibits transient responses. These transient responses are read out at the output layer via a linear weighted sum of the individual node states. The objective of RC is to implement a specific nonlinear transformation of the input signal or to classify the inputs. Classification involves the discrimination between a set of input data, for example, identifying features of images, voices, time series and so on. To perform its task, RC requires a training procedure. As recurrent networks are notoriously difficult to train, they were not widely used until the advent of RC. In RC, this problem is resolved by keeping the connections fixed. The only part of the system that is trained are the output layer weights. Thus, the training does not affect the dynamics of the reservoir itself. As a result of this training procedure, the system is capable to generalize, that is, process unseen inputs or attribute them to previously learned classes. Figure 1: Sketch of RC schemes. ( a ) Classical RC scheme. The input is coupled into the reservoir via a randomly connected input layer to the N nodes in the reservoir. The connections between reservoir nodes are randomly chosen and kept fixed, that is, the reservoir is left untrained. The reservoir's transient dynamical response is read out by an output layer, which are linear weighted sums of the reservoir node states x i ( t ). The output thus has the form . The coefficients w i of the sum are optimized in the training procedure to best project onto the target classes. ( b ) Scheme of RC utilizing a nonlinear node with delayed feedback. A reservoir is obtained by dividing the delay loop into N intervals and using time multiplexing. The input states are sampled and held for a duration τ , where τ is the delay in the feedback loop. For any time t 0 , the input state is multiplied with a mask, resulting in a temporal input stream J ( t ) that is added to the delayed state of the reservoir x ( t − τ ) and then fed into the nonlinear node. The output nodes are linear weighted sums of the tapped states in the delay line given by . ( c ) Scheme of the input data preparation and masking procedure. A time-continuous input stream u ( t ) or time-discrete input u ( k ) undergoes a sample and hold operation, resulting in a stream I ( t ) that is constant during one delay interval τ before it is updated. The random matrix M defines the coupling weights from the input layer to the virtual nodes. The temporal input sequence, feeding the input stream to the virtual nodes, is then given by J ( t )= M × I ( t ). Full size image To efficiently solve its tasks, a reservoir should satisfy several key properties. First, it should nonlinearly transform the input signal into a high-dimensional state space in which the signal is represented. This is achieved through the use of a large number of reservoir nodes that are connected to each other through the recurrent nonlinear dynamics of the reservoir. In practice, traditional RC architectures employ several hundreds/thousands of nonlinear reservoir nodes to obtain good performance. 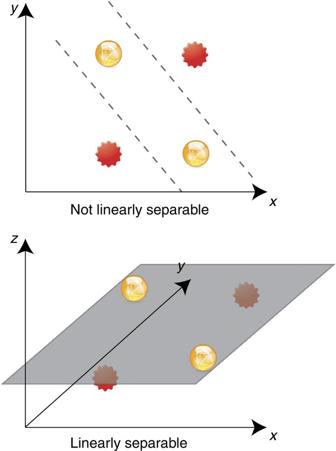Figure 2: Illustration of linear separability. It is well known that a non linear mapping from a small dimensional space into a high-dimensional space facilitates classification. This is illustrated in a simple example: In (a) a two-dimensional input space is depicted, in which the yellow spheres and the red stars cannot be separated with a single straight line. With a nonlinear mapping into a three-dimensional space, as depicted in (b), the spheres and stars can be separated by a single linear hyperplane. It can be shown that the higher dimensional the space is, the more likely it is that the data become linearly separable, see for example, ref.14. RC implements this idea: the input signal is nonlinearly mapped into the high-dimensional reservoir state through the transient response of the reservoir. Furthermore, in RC the output layer is a linear combination with adjustable weights of the internal node states. The readout and classification is thus realized with linear hyperplanes, as in the figure. In Figure 2 , we illustrate how such a nonlinear mapping to a high-dimensional state space facilitates separation (classification) of states [14] . Second, the dynamics of the reservoir should be such that it exhibits a fading memory (that is, a short-term memory): the reservoir state is influenced by inputs from the recent past, but independent of the inputs from the far past. This property is essential for processing temporal sequences (such as speech) for which only the recent history of the signal is important. Additionally, the results of RC computations must be reproducible and robust against noise. For this, the reservoir should exhibit sufficiently different dynamical responses to inputs belonging to different classes. At the same time, the reservoir should not be too sensitive: similar inputs should not be associated to different classes. These competing requirements define when a reservoir performs well. Typically, reservoirs depend on a few parameters (such as the feedback gain and so on) that must be adjusted to satisfy the above constraints. Experience shows that these requirements are satisfied when the reservoir operates (in the absence of input) in a stable regime, but not too far from a bifurcation point. Further introduction to RC, and in particular its connection with other approaches to machine learning, can be found in the Supplementary Discussion . Figure 2: Illustration of linear separability. It is well known that a non linear mapping from a small dimensional space into a high-dimensional space facilitates classification. This is illustrated in a simple example: In ( a ) a two-dimensional input space is depicted, in which the yellow spheres and the red stars cannot be separated with a single straight line. With a nonlinear mapping into a three-dimensional space, as depicted in ( b ), the spheres and stars can be separated by a single linear hyperplane. It can be shown that the higher dimensional the space is, the more likely it is that the data become linearly separable, see for example, ref. 14 . RC implements this idea: the input signal is nonlinearly mapped into the high-dimensional reservoir state through the transient response of the reservoir. Furthermore, in RC the output layer is a linear combination with adjustable weights of the internal node states. The readout and classification is thus realized with linear hyperplanes, as in the figure. Full size image In this article, we propose to implement a reservoir computer in which the usual structure of multiple connected nodes is replaced by a dynamical system comprising a nonlinear node subjected to delayed feedback. Mathematically, a key feature of time-continuous delay systems is that their state space becomes infinite dimensional. This is because their state at time t depends on the output of the nonlinear node during the continuous time interval [ t – τ , t [, with τ being the delay time. The dynamics of the delay system remains finite dimensional in practice [15] , but exhibits the properties of high dimensionality and short-term memory. Therefore, delay systems fulfil the demands required of reservoirs for proper operation. Moreover, they seem very attractive systems to implement RC experimentally, as only few components are required to build them. Here we show that this intuition is correct. Excellent performance on benchmark tasks is obtained when the RC paradigm is adapted to delay systems. This shows that very simple dynamical systems have high-level information-processing capabilities. Delay systems as reservoir In this section, we present the conceptual basis of our scheme, followed by the main results obtained for the two tasks we considered: spoken digit recognition and dynamical system modelling. We start by presenting in Figure 1b the basic principle of our scheme. Within one delay interval of length τ , we define N equidistant points separated in time by θ = τ / N . We denote these N equidistant points as 'virtual nodes', as they have a role analogous to the one of the nodes in a traditional reservoir. The values of the delayed variable at each of the N points define the states of the virtual nodes. These states characterize the transient response of our reservoir to a certain input at a given time. The separation time θ among virtual nodes has an important role and can be used to optimize the reservoir performance. We chose θ < T , with T being the characteristic time scale of the nonlinear node. With this choice, the states of the virtual nodes become dependent on the states of neighbouring nodes. Interconnected in this way, the virtual nodes emulate a network serving as reservoir ( Supplementary Discussion ). We demonstrate in the following that the single nonlinear node with delayed feedback performs comparably to traditional reservoirs. The virtual nodes are subjected to the time-continuous input stream u ( t ) or time-discrete input u ( k ) which can be a time-varying scalar variable or vector of any dimension Q . The feeding to the individual virtual nodes is achieved by serializing the input using time multiplexing. For this, the input stream u ( t ) or u ( k ) undergoes a sample and hold operation to define a stream I ( t ) that is constant during one delay interval τ , before it is updated. Thus, in our approach, the input to the reservoir is always discretized in time, no matter whether it stems from a time-continuous or time-discrete input stream. To define the coupling weights from the stream I ( t ) to the virtual nodes we introduce a random (NxQ) matrix M , in the following called mask (we recall that N is the number of virtual nodes). On carrying out the multiplication J ( t 0 )= M × I ( t 0 ) at a certain time t 0 , we obtain a N dimensional vector J ( t 0 ) that represents the temporal input sequence within the interval [ t 0 , t 0 + τ ]. Each virtual node is updated using the corresponding component of J ( t 0 ). Alternatively, one can view J ( t ) as a continuous time scalar function that is constant over periods, corresponding to the separation θ of the virtual nodes. Figure 1c illustrates the above input preparation and masking procedure. After a period τ , the states of all virtual nodes have been updated and the new reservoir state is obtained. Subsequently, I ( t 0 ) is updated to drive the reservoir during the next period of duration τ . For each period τ , the reservoir state is read out for further processing. A training algorithm assigns an output weight to each virtual node, such that the weighted sum of the states approximates the desired target value as closely as possible (see Supplementary discussion ). The training of the read-out follows the standard procedure for RC [5] , [7] . The testing is then performed using previously unseen input data of the same kind of those used for training. To demonstrate our concept, we have chosen the widely studied Mackey–Glass oscillator [16] . The model of this dynamical system with its characteristic delayed feedback term, extended to include the external input J ( t ), reads with X denoting the dynamical variable, its derivative with respect to a dimensionless time t , and τ the delay in the feedback loop. The characteristic time scale of the oscillator, determining the decay of X in the absence of the delayed feedback term, has been normalized to T =1. The parameters η and γ represent feedback strength and input scaling, respectively. The value of η we use guarantees that the system operates in a stable fixed point in the absence of external input ( γ =0). With input, however, the system might exhibit complex dynamics. The choice of the nonlinearity in equation (1) has two main advantages. First, it can be easily implemented by an analogue electronic circuit [17] , which allows for fine parameter tuning [18] . This is the physical realization we have employed for the experimental demonstration ( Fig. 3) . Second, the exponent p can be used to tune the nonlinearity if needed. However, we expect other nonlinear functions to perform equally well. 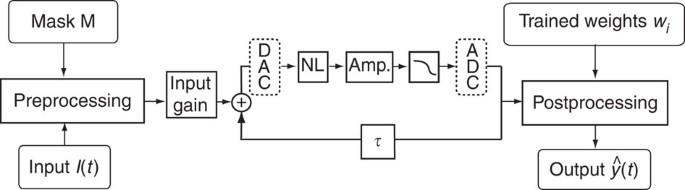Figure 3: Schematic of the experimental reservoir computer. The Mackey–Glass type nonlinear node is realized as in ref.17. The time constant of the system isT=10 ms. The delay loop is implemented digitally by means of Analog to Digital and Digital to Analog Converters (ADC and DAC). The preprocessing to create the input streamγJ(t), withγthe adjustable input gain described in equation (1), and the postprocessing to create the outputare also realized digitally. SeeSupplementary discussionfor further details on the experimental implementation. Figure 3: Schematic of the experimental reservoir computer. The Mackey–Glass type nonlinear node is realized as in ref. 17 . The time constant of the system is T =10 ms. The delay loop is implemented digitally by means of Analog to Digital and Digital to Analog Converters (ADC and DAC). The preprocessing to create the input stream γJ ( t ), with γ the adjustable input gain described in equation (1), and the postprocessing to create the output are also realized digitally. See Supplementary discussion for further details on the experimental implementation. Full size image Spoken digit recognition task We now demonstrate by experiment and simulation, the capability of our single nonlinear delay-dynamical node to perform isolated spoken digits recognition. The isolated spoken digit recognition task, as introduced by Doddington and Schalk [19] , is generally accepted as a benchmark speech recognition task. Our experimental realization has a Mackey–Glass nonlinearity with an exponent of p =7 that is easily obtained with standard electronic components. We have verified through numerical simulations that a broad range of values of p yields similar results. The virtual node separation is set at θ =0.2 that offers optimal performance (Methods section), whereas the total number of virtual nodes is N =400. The specifics of the training procedure are detailed in the Supplementary Discussion and the Methods section. 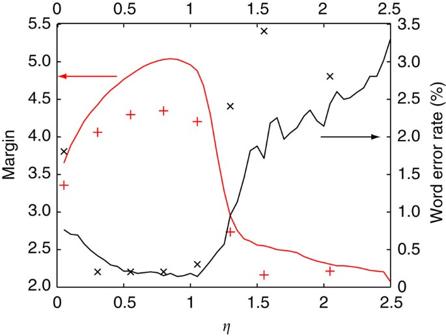Figure 4: Numerical and experimental results for spoken digit recognition. They-axis on the left-hand side denotes the margin, whereas they-axis on the right-hand side denotes the word error rate. The abscissa represents the parameterη.γhas been kept fixed at 0.5 and the exponent is set top=7. The delay time is set atτ=80, withN=400 neurons ofθ=0.2 separation. The red line represents results for the numerically obtained margin and the black line represents the numerically obtained word error rate. The red and black crosses denote the corresponding experimental results. As an example, Figure 4 depicts the experimentally and numerically obtained classification performance of unknown samples as a function of η for γ =0.5, which has been chosen such that input and feedback signals are of the same order of magnitude. The classification performance is expressed in two ways: the word error rate (WER) that shows the percentage of words that have been wrongly classified, and the margin (distance) between the reservoir's best guess of the target and the closest competitor. It can be seen that an increase in margin corresponds to a decrease in WER. Our results show that there is a broad parameter range in η with good performance, with an optimum for both, margin and WER, around η =0.8. Note that the performance breaks down when η approaches 1. This is expected as it corresponds to the threshold of instability of the MG oscillator when there is no input ( γ =0). At the optimum value of η , we obtain a WER as low as 0.2% in experiments and 0.14% in numerical simulations. This corresponds to only one misclassification in 500 words. These performance levels are comparable to or even better than those obtained with traditional RC composed of more than 1,200 nodes for which a WER of 4.3% was reported [11] , with a reservoir of 308 nodes for which more recently a WER of 0.2% was obtained [12] and also with alternative approaches based on hidden Markov models that achieved a WER of 0.55% (ref. 20 ). Figure 4: Numerical and experimental results for spoken digit recognition. The y -axis on the left-hand side denotes the margin, whereas the y -axis on the right-hand side denotes the word error rate. The abscissa represents the parameter η . γ has been kept fixed at 0.5 and the exponent is set to p =7. The delay time is set at τ =80, with N =400 neurons of θ =0.2 separation. The red line represents results for the numerically obtained margin and the black line represents the numerically obtained word error rate. The red and black crosses denote the corresponding experimental results. Full size image NARMA task as an example of dynamical system modelling We now present results from numerical simulations demonstrating the computational capabilities of the single nonlinear delay-dynamical node for a second task, commonly used in RC literature: dynamical system modelling, in particular training the readout to reproduce a certain signal [21] , [22] . Specifically, we train the system to model the response to white noise of a discrete-time tenth order nonlinear auto-regressive moving average (NARMA) system, originally introduced in reference 23 . The details of this benchmark are described in the Supplementary Discussion and in the Methods section. To quantify the performance of the reservoir, the normalized root mean square error (NRMSE) of the predicted value versus the value obtained from the NARMA model is used. Up to now, the best performance reported in traditional RC for a reservoir of N =100 nodes, is NRMSE=0.18 (ref. 12 ). If the reservoir is replaced by a shift register that contains the input, the minimal NRMSE is 0.4. NRMSE values below this level require a nonlinear reservoir. We have chosen a nonlinear exponent of p =1, resulting in a weak nonlinearity that allows for longer memory as compared with the previously used value of p =7 ( Supplementary Discussion ). 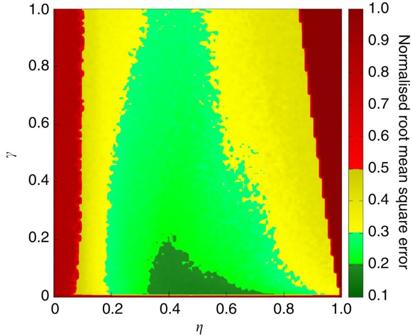Figure 5: Simulation results for the NARMA task. The two scanned parameters areγ(input scaling) andη(feedback strength). The exponent in equation (1) is set top=1. Other characteristics of the reservoir are as inFigure 4(τ=80,N=400,θ=0.2). The obtained performance for the NARMA-10 task, expressed as a normalized root mean square error, is encoded in colour. Figure 5 depicts our numerical results in the γ − η plane. A large region with NRMSE<0.2 (dark green) has been obtained. 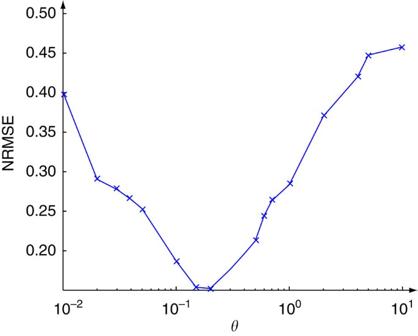Figure 6: Performance of NARMA task as a function of node separation. Plot of the normalized NRMSE for the NARMA-10 task (simulations) versus the separationθof the virtual nodes. Parameters are:η=0.5,γ=0.05,p=1,τ=400θ. In Figure 6, we depict the NRMSE as a function of the virtual node separation θ . The optimal value lies around θ =0.2. When θ is larger, there is not enough coupling between virtual nodes, and performance decreases. When θ is smaller, too much averaging causes decreased performance. The minimal normalized root mean square error is as low as NRMSE=0.15. We therefore achieved comparable performance to conventional RC, but with a much simpler architecture. Figure 5: Simulation results for the NARMA task. The two scanned parameters are γ (input scaling) and η (feedback strength). The exponent in equation (1) is set to p =1. Other characteristics of the reservoir are as in Figure 4 ( τ =80, N =400, θ =0.2). The obtained performance for the NARMA-10 task, expressed as a normalized root mean square error, is encoded in colour. Full size image Figure 6: Performance of NARMA task as a function of node separation. Plot of the normalized NRMSE for the NARMA-10 task (simulations) versus the separation θ of the virtual nodes. Parameters are: η =0.5, γ =0.05, p =1, τ =400 θ . Full size image We have demonstrated, both in experiment and simulation, that a simple nonlinear dynamical system subject to delayed feedback can efficiently perform information processing. As a consequence, our simple scheme can replace the complex networks used in traditional RC. Moreover, to the best of our knowledge, this experiment represents the first hardware implementation of RC with results comparable to those obtained with state-of-the-art digital realizations ( Supplementary Discussion ). To get good performance with our system, a number of parameters need to be adjusted. These include the feedback gain η , the input gain γ , the delay time τ , the separation of virtual nodes in the delay line θ , the type of nonlinearity (in our case the exponent p of the MG system), and the choice of input mask. These parameters have analogues with similar parameters used in traditional RC: feedback gain and input gain have similar roles to spectral radius and input scaling; the delay time τ is related to the number of nodes and the separation of the virtual nodes to the sparsity of the interconnection matrix; the type of nonlinearity can also be varied in traditional RC and so on. As demonstrated here, some of the parameters can vary significantly around certain optimal values and still yield very good results. As experience with systems such as ours grows, we expect–as in traditional RC–that good heuristics on what parameter values to use will emerge. We expect that delay reservoirs can be realized that are, within some restrictions, versatile for different tasks. Moreover, owing to their much simpler hardware implementation, specifically optimized solutions for certain tasks could make sense. From a fundamental point of view, the simplicity of our architecture should facilitate gaining a deeper understanding of the interplay of dynamical properties and reservoir performance. Besides the fundamental aspect of understanding information processing capabilities of dynamical systems, our architecture also offers practical advantages. The reduction of a complex network to a single hardware node facilitates implementations enormously, because only few components are needed. Nevertheless, the use of delay dynamical systems implies certain constraints, because the feeding of the virtual nodes is carried out serially, in contrast to the parallel feeding of the nodes in traditional RC. This serial feeding procedure results in a slow-down of the information processing, compared with parallel feeding. This potential slow-down is compensated for by the much simpler hardware architecture of the reservoir, and by the fact that the read-out can be taken at a single point of the delay line. These simplifications will enable ultra-high-speed implementations, using high-speed components that would be too demanding or expensive to be used for many nodes. In particular, realizations based on electronics or photonics systems should be feasible using this simple scheme, including real-time processing capabilities. Moreover, we expect that compromises can be found concerning speed, performance and memory capacity by extending the concept to network motifs of delay-coupled elements. Ultimately, a novel information-processing paradigm might emerge. Spoken digit recognition task In the spoken digit recognition task, the input dataset consists of a subset of the NIST TI-46 corpus [24] with ten spoken digits (0–9), each one recorded ten times by five different female speakers. Hence, we have 500 spoken words, all sampled at 12.5 kHz. The input u ( k ) (with k the discretized time) for the reservoir is, in this case, a set of 86-dimensional state vectors (channels) with up to 130 time steps. Each of these inputs represents a spoken digit, preprocessed using a standard cochlear ear model [25] . To construct an appropriate target function, ten linear classifiers are trained, each representing a different digit of the dataset. The target function is −1 if the spoken word does not correspond to the sought digit, and +1 if it does. For every target, the time trace is averaged in time and a winner-takes-all approach is applied to select the actual digit. To eliminate the impact of the specific division of the available data samples between regularization, training and testing, we used n -fold cross-validation. This means that the entire process of regularization, training and testing is repeated n times (with n =20) on the same data, but each time with a different assignment of data samples to each of the three stages. The reported performances are the mean across these n runs. For the spoken digit recognition task, the mask consists of a random assignment of three values: 0.59, 0.41 and 0. The first two values have equal probability of being selected, whereas the third one is more likely to be selected. Using a zero mask value implies that some nodes are insensitive to certain channels, thus avoiding averaging of all the channels. NARMA10 task The NARMA10 task is one of the most widely used benchmarks in RC. It was introduced in [21] , and used in many other publications in the context of RC, for instance in references 23 , 26 . For the NARMA10 task, the input u ( k ) of the system consists of scalar random numbers, drawn from a uniform distribution in the interval [0, 0.5] and the target y ( k +1) is given by the following recursive formula The input stream J ( t ) for the NARMA10 test is obtained from u k according to the procedure discussed in the manuscript. For the regularization, training and test of the dynamical system modelling task, we used 4 samples with a length of 800 points each and twofold cross-validation. The input scaling for the mask consists of a random series of amplitudes of 0.1 and −0.1. The input signal, multiplied with the mask and the input scaling factor γ, feeds the Mackey-Glass node as in equation (1). The importance of the parameters γ, the feedback strength η, and the separation between virtual nodes θ , has been discussed above. In particular, θ has a crucial role. In Figure 6, we show the numerically obtained performance of the Mackey–Glass system for the NARMA10 test when scanning θ . The optimal point is found for virtual node separations of θ =0.2, in units of the characteristic time scale of the nonlinear node. For shorter separations, too much averaging takes place and the Mackey–Glass system does not respond to the external input. For larger separations, the connectivity among virtual nodes is lost and, consequently, also the memory with respect to previous input. For node separations θ >3, the NRMSE reaches a level of 0.4, which is the performance of a shift-register. How to cite this article: Appeltant, L. et al . Information processing using a single dynamical node as complex system. Nat. Commun. 2:468 doi: 10.1038/ncomms1476 (2011).